An alternative pathway contributes to phenylalanine biosynthesis in plants via a cytosolic tyrosine:phenylpyruvate aminotransferase Phenylalanine is a vital component of proteins in all living organisms, and in plants is a precursor for thousands of additional metabolites. Animals are incapable of synthesizing phenylalanine and must primarily obtain it directly or indirectly from plants. Although plants can synthesize phenylalanine in plastids through arogenate, the contribution of an alternative pathway via phenylpyruvate, as occurs in most microbes, has not been demonstrated. Here we show that plants also utilize a microbial-like phenylpyruvate pathway to produce phenylalanine, and flux through this route is increased when the entry point to the arogenate pathway is limiting. Unexpectedly, we find the plant phenylpyruvate pathway utilizes a cytosolic aminotransferase that links the coordinated catabolism of tyrosine to serve as the amino donor, thus interconnecting the extra-plastidial metabolism of these amino acids. This discovery uncovers another level of complexity in the plant aromatic amino acid regulatory network, unveiling new targets for metabolic engineering. Aromatic amino acids are essential constituents of proteins in all living organisms, whereas in plants, phenylalanine (Phe) and tyrosine (Tyr) also serve as precursors for thousands of vital and specialized compounds. Approximately 20–30% of photosynthetically fixed carbon is directed towards synthesis of phenylalanine, and in turn to lignin [1] , the central structural component of plant cell walls and the major impediment to cellulosic biofuel production. In addition to structural roles, phenylalanine-derived compounds function in plant defence and ultraviolet protection (for example, flavonoids and various phenolics) [2] , [3] , signalling (for example, isoflavonoids) [4] and reproduction (for example, anthocyanins and phenylpropanoid/benzenoid volatiles) [3] . Moreover, tyrosine-derived metabolites, such as tocopherols (vitamin E) [5] , plastoquinone [6] , cyanogenic glycosides [7] and suberin [8] have crucial roles in plant fitness. Phenylalanine and tyrosine are synthesized from chorismate, the final product of the shikimate pathway [9] , [10] , which is converted by chorismate mutase to prephenate. Subsequent conversion of prephenate to phenylalanine and tyrosine occurs through alternative routes. In the first (the arogenate pathway), a shared transamination reaction catalysed by prephenate aminotransferase (PPA-AT), produces L -arogenate, which can then either be dehydrated/decarboxylated to phenylalanine by arogenate dehydratase (ADT) or dehydrogenated/decarboxyled to tyrosine by arogenate dehydrogenase (ADH; Fig. 1 ). In the other routes (the phenylpyruvate/4-hydroxyphenylpyruvate pathways), these reactions occur in reverse order: prephenate is first subjected to dehydration/decarboxylation or dehydrogenation/decarboxylation to form phenylpyruvate or 4-hydroxyphenylpyruvate, respectively. Then the corresponding products undergo transamination to phenylalanine and tyrosine ( Fig. 1 ). Most microorganisms appear to utilize only the phenylpyruvate/4-hydroxyphenylpyruvate pathways [11] , [12] , [13] , with a few exceptions [14] . In contrast, phenylalanine and tyrosine biosynthesis in plants has only been described to occur via the arogenate pathway [15] , [16] , [17] , [18] . Nevertheless, overexpression of a bacterial bifunctional chorismate mutase/prephenate dehydratase ( PheA ) in Arabidopsis resulted in significantly increased phenylalanine production [19] , implicating the presence of an aminotransferase capable of converting phenylpyruvate to phenylalanine in plants, as it occurs in the final step of the microbial phenylpyruvate pathway. Although several plant aminotransferases, mainly participating in aromatic amino-acid catabolism, have recently been described [20] , [21] , [22] , [23] , none of them have been demonstrated to function in phenylalanine biosynthesis. 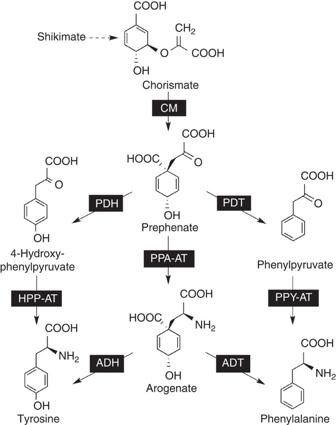Figure 1: Proposed phenylalanine and tyrosine biosynthetic pathways in plants. ADH, arogenate dehydrogenase; ADT, arogenate dehydratase; CM, chorismate mutase; HPP-AT, 4-hydroxyphenylpyruvate aminotransferase; PDH, prephenate dehydrogenase; PDT, prephenate dehydratase; PPA-AT, prephenate aminotransferase; PPY-AT, phenylpyruvate aminotransferase. Figure 1: Proposed phenylalanine and tyrosine biosynthetic pathways in plants. ADH, arogenate dehydrogenase; ADT, arogenate dehydratase; CM, chorismate mutase; HPP-AT, 4-hydroxyphenylpyruvate aminotransferase; PDH, prephenate dehydrogenase; PDT, prephenate dehydratase; PPA-AT, prephenate aminotransferase; PPY-AT, phenylpyruvate aminotransferase. Full size image Previously we demonstrated that PhADT1 downregulation in Petunia hybrida flowers, which emit high levels of phenylalanine-derived volatiles [24] , [25] , resulted in a greater decrease in phenylalanine levels compared with the effect of PhPPA-AT downregulation (up to 82% versus 20% reduction, respectively) [16] , [17] . Such a differential impact on phenylalanine levels from the downregulation of these individual genes was suggested to be due to either sufficient residual PPA-AT activity in the PhPPA-AT RNAi lines capable of sustaining the arogenate pathway, or the redirection of carbon flux from accumulated prephenate in the PhPPA-AT RNAi lines through the hitherto undetected alternative phenylpyruvate pathway [17] . Here to test these hypotheses, we generated RNAi transgenic petunia plants in which both PhADT1 and PhPPA-AT genes were simultaneously downregulated. If the phenylalanine and volatile phenotypes in PhADT1 plants can be rescued by concurrent downregulation of PhPPA-AT , this would be consistent with redirection of flux from prephenate through an alternative pathway. Indeed, detailed metabolic profiling of PhADT1xPhPPA-AT RNAi lines provides evidence in agreement with the involvement of an alternative pathway. To provide further support, we identify a petunia phenylpyruvate aminotransferase gene (designated as PhPPY-AT), downregulation of which leads to reduction of phenylalanine and phenylalanine-derived scent compounds. Extensive biochemical characterization of PhPPY-AT reveals that it preferentially converts phenylpyruvate to phenylalanine, and unexpectedly strongly favours tyrosine as the amino donor. In addition, feeding experiments with petunia petals show that the 15 N label from supplied 15 N-tyrosine is retrieved in phenylalanine, and higher phenylalanine labelling occurs in PhADT1xPhPPA-AT RNAi lines than in wild-type, consistent with higher flux through the phenylpyruvate pathway when the flux into the arogenate pathway is limiting. Moreover, we have shown that PhPPY-AT is a cytosolic enzyme, and when the tyrosine pool is reduced via overexpression of a cytosolic tyrosine decarboxylase, it leads to a decrease in phenylalanine levels. Taken together, these results demonstrate for the first time that the microbial-like phenylpyruvate pathway operates in plants, phenylalanine biosynthesis is not limited to plastids, and that there is an interconnection between aromatic amino-acid catabolism and biosynthesis in planta . PhPPA- AT suppression in PhADT1 RNAi lines rescues Phe levels To determine if phenylpyruvate can serve as an intermediate in phenylalanine biosynthesis in petunia, 2 days old wild-type flowers were fed with 10 mM L -[ring- 2 H 5 ]-phenylpyruvate for 6 h during the night. Indeed, time-of-flight (TOF) Liquid chromatography-mass spectrometry (LC-MS) analysis revealed that phenylalanine was labelled up to 9%. Next, to examine the contribution of the undiscovered phenylpyruvate pathway towards phenylalanine biosynthesis in petunia flowers, PhADT1 and PhPPA-AT RNAi lines were crossed to simultaneously downregulate both steps in the arogenate pathway. Five independent lines (A–E) were generated and found to display comparable degrees of PhADT1 and PhPPA-AT mRNA suppression to those in the parental lines ( Fig. 2a,b ). Phenylalanine levels in all five PhADT1xPhPPA-AT RNAi lines were rescued, not just to PhPPA-AT RNAi levels, but surprisingly to that of wild-type ( Fig. 2c ), consistent with the hypothesized redirection of flux through an alternative pathway. One independent line (A) was selected for further biochemical analysis and metabolic profiling of emitted floral volatiles as well as internal pools of intermediates and end products. Similar to expression levels, ADT and PPA-AT activities, in the flowers of the PhADT1xPhPPA-AT RNAi line A resembled the parents, while metabolic profiling revealed that similar to the PhPPA-AT RNAi line, prephenate and arogenate accumulated, while tyrosine, tryptophan, and shikimate levels matched the wild type ( Supplementary Fig. S1 ). Moreover, like phenylalanine levels, phenylalanine-derived volatiles were rescued to those of wild type ( Fig. 2c , Supplementary Fig. S1 and Supplementary Table S1 ). Feeding petunia petals from PhADT1xPhPPA-AT RNAi flowers with 10 mM 2 H 5 -phenylpyruvate resulted in labelling of the phenylalanine pool by 24% (2.7-fold higher than wild type), further supporting the hypothesized increased flux through an alternative pathway when the arogenate route is limiting. 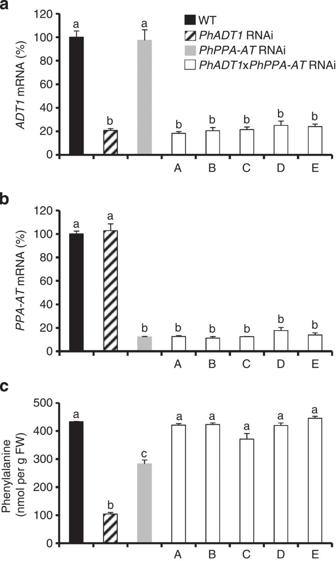Figure 2: Effect of downregulatingPhPPA-ATin thePhADT1RNAi line on phenylalanine levels in petunia flowers. The levels ofPhADT1mRNA (a) andPhPPA-ATmRNA (b) were determined by qRT–PCR, and phenylalanine pools (c) were determined by GC-MS in petals of wild-type (WT; black), thePhADT1RNAi line (striped), thePhPPA-ATRNAi line (grey) and five independentPhADT1xPhPPA-ATRNAi lines (A–E, white) petunia flowers harvested at 20:00 h, 2 days postanthesis. Data are means±s.e.m. (n=5 biological replicates). Columns with the same letters above are not significantly different based on Tukey’s test (P<0.05; one-way ANOVA). Figure 2: Effect of downregulating PhPPA-AT in the PhADT1 RNAi line on phenylalanine levels in petunia flowers. The levels of PhADT1 mRNA ( a ) and PhPPA-AT mRNA ( b ) were determined by qRT–PCR, and phenylalanine pools ( c ) were determined by GC-MS in petals of wild-type (WT; black), the PhADT1 RNAi line (striped), the PhPPA-AT RNAi line (grey) and five independent PhADT1 x PhPPA-AT RNAi lines (A–E, white) petunia flowers harvested at 20:00 h, 2 days postanthesis. Data are means±s.e.m. ( n =5 biological replicates). Columns with the same letters above are not significantly different based on Tukey’s test ( P <0.05; one-way ANOVA). Full size image PhPPY-AT prefers phenylpyruvate and Tyr as substrates Although most microorganisms utilize the phenylpyruvate route to synthesize phenylalanine [11] , [12] , [13] , they rely on multiple functionally redundant aminotransferases with broad substrate specificity to convert phenylpyruvate to phenylalanine [26] . As aminotransferase reactions are reversible in nature, we therefore used the Cucumis melo L., Cucurbitaceae enzyme CmArAT1 (ADC45389.1), which catalyses the catabolism of phenylalanine to phenylpyruvate for production of melon fruit scent compounds [20] , as query for a tBlastn search against our petunia RNA-seq database to identify a candidate phenylpyruvate aminotransferase (PPY-AT). The top hit in the tBLASTn search ( E -value < e −170 ) revealed a contig representing a full-length mRNA encoding a protein, later designated as the PhPPY-AT, of 447 amino acids sharing 66% identity/82% similarity to CmArAT1. To examine if PhPPY-AT is capable of converting phenylpyruvate to phenylalanine, we initially assessed its ability to functionally complement the Escherichia coli ( E . coli ) phenylalanine auxotrophic mutant DL39 (ref. 27 ). This mutant lacks the three aminotransferases, AspC (aspartate aminotransferase), TyrB (L-Tyrosine aminotransferase) and IlvE (branched-chain aminotransferase), shown to participate in phenylalanine and tyrosine biosynthesis. The PhPPY-AT open reading frame, subcloned in the arabinose-inducible vector pBad33 (ref. 28 ) and introduced into the DL39 mutant, restored the ability of the mutant to grow in the absence of exogenously supplied phenylalanine and tyrosine ( Supplementary Fig. S2a ). Moreover, in vitro enzyme assays using crude extracts from the DL39 mutant expressing PhPPY-AT in the presence of phenylpyruvate, glutamate as an amino donor and the pyridoxal phosphate cofactor, confirmed that PhPPY-AT transaminates phenylpyruvate to phenylalanine ( Supplementary Fig. S2b ). For biochemical characterization of the isolated PhPPY-AT, its coding region was expressed in E. coli as an inducible fusion protein containing a hexahistidine tag, which was subsequently removed before analysis. Out of the 19 common L-amino acids (except phenylalanine, the product of the reaction) tested as amino donors, tyrosine by far most efficiently supplied the amino group for the conversion of phenylpyruvate to phenylalanine, whereas PPY-AT activities with glutamate, methionine and leucine did not exceed 13% of the activity with tyrosine ( Supplementary Table S2 ). Of the five keto acids tested in the presence of tyrosine, only phenylpyruvate and α-ketoglutarate effectively served as substrates, and no activity was detected with prephenate ( Supplementary Table S3 ), the substrate of PhPPA-AT [17] . Similarly, with glutamate as the amino donor, phenylpyruvate was the best substrate and again no activity was detected with prephenate ( Supplementary Table S3 ), indicating that PhPPY-AT does not moonlight in the arogenate pathway. Apparent K m values of PhPPY-AT for phenylpyruvate were 1.5 and 2.6 mM when tested with tyrosine and glutamate, respectively, as amino donors, whereas K m values for tyrosine and glutamate in the presence of phenylpyruvate were 1.9 and 11.1 mM, respectively ( Table 1 ). Catalytic efficiencies ( k cat /K m ) for phenylpyruvate and tyrosine were comparable (0.965 and 0.769 mM −1 s −1 ) when used together. However, when tyrosine was substituted by glutamate the catalytic efficiency of PhPPY-AT for phenylpyruvate was reduced by half (0.461 mM −1 s −1 ), and that for the amino donor (glutamate) was reduced by 20-fold (0.039 mM −1 s −1 ; Table 1 ). Table 1 Kinetic parameters of PhPPY-AT. Full size table PhPPY-AT also catalysed the reverse reactions, conversion of phenylalanine to phenylpyruvate using 4-hydroxyphenylpyruvate or α-ketoglutarate as amino acceptors ( Table 1 ). The forward and reverse reactions with glutamate and α-ketoglutarate, respectively, occurred with similar catalytic efficiencies ( Table 1 ). However, catalytic efficiencies of the reverse reaction using 4-hydroxyphenylpyruvate and phenylalanine as substrates (0.089 and 0.039 mM −1 s −1 , respectively) were 11- and 20-fold lower than that in the forward reaction for phenylpyruvate (0.965 mM −1 s −1 ) and tyrosine (0.769 mM −1 s −1 ), respectively ( Table 1 ). As the reverse reaction with 4-hydroxyphenylpyruvate leads to tyrosine formation, we checked whether phenylalanine is the best amino donor. Indeed, phenylalanine showed the highest activity with 4-hydroxyphenylpyruvate as amino acceptor, although glutamate, methionine and leucine displayed comparable activities ( Supplementary Table S2 ). PhPPY-AT is localized in the cytosol In plants phenylalanine biosynthesis via the arogenate pathway takes place in plastids [10] , [16] , [18] , [29] , [30] . Surprisingly however, the protein targeting prediction programs (WolfPSort: http://wolfpsort.org/ [31] ; Predotar: http://urgi.versailles.inra.fr/predotar/predotar.html [32] ; TargetP: http://www.cbs.dtu.dk/services/TargetP/ [33] ) revealed the absence of an N-terminal transit peptide for plastidic localization in the PhPPY-AT protein. To experimentally determine PhPPY-AT subcellular localization, the complete coding region of the gene was fused to either the 5′- or 3′-ends of a green fluorescent protein (GFP) reporter gene. The resulting constructs were transferred to Arabidopsis protoplasts and the corresponding transient GFP expression was analysed by confocal microscopy ( Fig. 3 ). Independent of PhPPY-AT position, GFP fluorescence was detected only in the cytosol ( Fig. 3a,b ), similar to protoplasts expressing GFP alone ( Fig. 3c ), and did not overlap with autofluorescence of chloroplasts or GFP fused to the transit peptide of ribulose-1,5-bis-phosphate carboxylase/oxigenase (Rubisco) small subunit ( Fig. 3d ). To biochemically confirm the cytosolic localization of PhPPY-AT, its activity was assayed in cytosolic and plastidial fractions prepared from wild-type petunia petals [34] , [35] ( Table 2 ). Indeed, the cytosolic fraction showed 2.5-fold enrichment in PhPPY-AT activity, similar to the 2.6-fold enrichment in the activity of the cytosolic marker alcohol dehydrogenase, relative to crude extract. At the same time, no enrichment in activity of the plastidic marker, PPA-AT, was detected in this fraction ( Table 2 ). In contrast, no PhPPY-AT nor alcohol dehydrogenase activities were detected in the plastidic fraction, which exhibited a 3-fold enrichment in PPA-AT activity compared with crude extract ( Table 2 ). Taken together these results demonstrate that PhPPY-AT is localized in the cytosol, not in plastids. 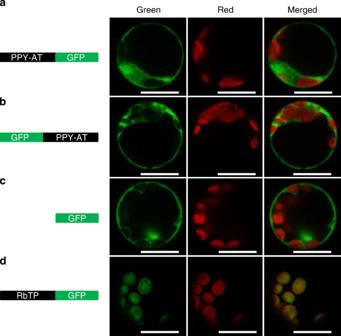Figure 3: Petunia PPY-AT is localized to the cytosol. Schematic diagrams of GFP-fusion constructs are shown on the left with corresponding transient expression inArabidopsisprotoplasts on the right. GFP fluorescence and chloroplast autofluorescence are shown in the green and red panels, respectively. The merged panel shows the overlay of the green and red fluorescence images. GFP alone and RbTP (Rubisco transit peptide)-GFP were used as cytosolic and plastidic markers, respectively. Scale bars, 50 μm. Figure 3: Petunia PPY-AT is localized to the cytosol. Schematic diagrams of GFP-fusion constructs are shown on the left with corresponding transient expression in Arabidopsis protoplasts on the right. GFP fluorescence and chloroplast autofluorescence are shown in the green and red panels, respectively. The merged panel shows the overlay of the green and red fluorescence images. GFP alone and RbTP (Rubisco transit peptide)-GFP were used as cytosolic and plastidic markers, respectively. Scale bars, 50 μm. Full size image Table 2 Enrichment of PPY-AT activity in cytosol. Full size table PhPPY-AT is involved in Phe biosynthesis in vivo Genes involved in biosynthesis of phenylalanine and phenylalanine-derived volatile compounds in petunia flowers typically display a spatial, temporal and rhythmic expression profile corresponding with floral volatile emission [16] , [17] , [25] , [34] , [35] , [36] . Thus, PhPPY-AT transcript levels were investigated by qRT–PCR with gene-specific primers. Although PhPPY-AT expression did not show a specific spatial profile or change over flower development, it did exhibit rhythmicity with maximum around 15:00 h, positively correlating with phenylalanine levels [16] and emission of phenylalanine-derived volatiles [24] , [25] over a daily light/dark cycle ( Supplementary Fig. S3 ). To further determine whether PhPPY-AT is involved in phenylalanine biosynthesis in planta , PhPPY-AT expression was transiently downregulated in flowers of wild-type petunia, the PhADT1xPhPPA-AT RNAi line, and the PhADT1 and PhPPA-AT RNAi parental lines by infiltrating agrobacteria carrying the PhPPY-AT RNAi construct. Approximately 70–75% reduced expression levels of PhPPY-AT were achieved in all lines relative to their corresponding controls 2 days after infiltration ( Fig. 4a ). Reduced PhPPY-AT expression led to a decrease in phenylalanine levels by 13% in wild-type flowers and by 28–33% in the PhADT1xPhPPA-AT RNAi ( Fig. 4a ) and parental RNAi lines ( Supplementary Fig. S4 ). Interestingly, downregulation of PhPPY-AT had a greater impact on phenylalanine-derived volatiles in the PhADT1xPhPPA-AT RNAi line compared with wild-type and the parental RNAi lines (64% versus 20–40%, respectively; Fig. 4a and Supplementary Fig. S4 ). Moreover, when PhPPY-AT was overexpressed in the wild-type and PhADT1xPhPPA-AT RNAi background, the levels of phenylalanine increased by 177% and 37%, respectively, and volatiles by 130% and 73%, respectively ( Fig. 4b ). Taken together, these results provide in vivo evidence that cytosolic PhPPY-AT is involved in phenylalanine formation. 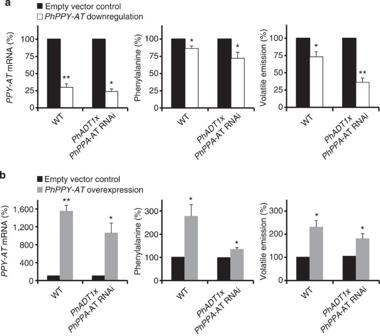Figure 4: Effect ofPhPPY-ATdownregulation and overexpression on Phe and Phe-derived volatile levels in petunia flowers. (a) Downregulation ofPhPPY-ATin petunia flowers (left panel) significantly decreases the levels of phenylalanine (middle panel) and phenylalanine-derived volatiles (right panel). For each genetic background, black and white columns represent flowers infiltrated with the empty vector or thePhPPY-ATRNAi construct, respectively. (b) Overexpression ofPhPPY-ATin petunia flowers (left panel) significantly increases the levels of phenylalanine (middle panel) and phenylalanine-derived volatiles (right panel). For each genetic background, black and grey columns represent flowers infiltrated with the empty vector or thePhPPY-AToverexpression construct, respectively. Foraandb, data are presented as a percentage relative to the corresponding empty-vector reference. Data are means±s.e.m. (n≥3 biological replicates). *P<0.05 and **P<0.01 as determined by paired two-tailed Student’st-tests. Figure 4: Effect of PhPPY-AT downregulation and overexpression on Phe and Phe-derived volatile levels in petunia flowers. ( a ) Downregulation of PhPPY-AT in petunia flowers (left panel) significantly decreases the levels of phenylalanine (middle panel) and phenylalanine-derived volatiles (right panel). For each genetic background, black and white columns represent flowers infiltrated with the empty vector or the PhPPY-AT RNAi construct, respectively. ( b ) Overexpression of PhPPY-AT in petunia flowers (left panel) significantly increases the levels of phenylalanine (middle panel) and phenylalanine-derived volatiles (right panel). For each genetic background, black and grey columns represent flowers infiltrated with the empty vector or the PhPPY-AT overexpression construct, respectively. For a and b , data are presented as a percentage relative to the corresponding empty-vector reference. Data are means±s.e.m. ( n ≥3 biological replicates). * P <0.05 and ** P <0.01 as determined by paired two-tailed Student’s t -tests. Full size image Tyr catabolism and Phe biosynthesis are interconnected Previously it has been shown that the transamination of prephenate to arogenate by PhPPA-AT in petunia depends exclusively on aspartate and glutamate as amino donors [17] . In contrast, biochemical characterization of PhPPY-AT has revealed that tyrosine is by far the most efficient amino donor ( Supplementary Table S2 ). To verify if tyrosine participates in the transamination of phenylpyruvate in vivo , feeding experiments with 15 N-tyrosine were performed with 2 day-old wild-type petunia flowers and the 15 N incorporation of the labelled amino group in phenylalanine was analysed. After 6 h of continuous feeding with 10 mM 15 N-tyrosine, the tyrosine pool was labelled by >87%, whereas the phenylalanine pool was labelled by 5% ( Fig. 5a ). All other amino acids remained unlabelled, with the exception of glutamate and aspartate, which were both labelled by <1.3% after 6 h. No labelling was retrieved in phenylalanine when ring-labelled 2 H 4 -tyrosine was supplied instead, confirming that tyrosine is not converted to phenylalanine via dehydration. When 10 mM 15 N-tyrosine was fed to flowers of the PhADT1xPhPPA-AT RNAi line, the phenylalanine pool was labelled ~52% higher than that detected in wild-type ( Fig. 5a ). Labelling experiments with the PhADT1 and PhPPA-AT parental RNAi lines showed 25% lower and 31% higher incorporation of 15 N label into phenylalanine than wild-type, respectively ( Fig. 5a ). 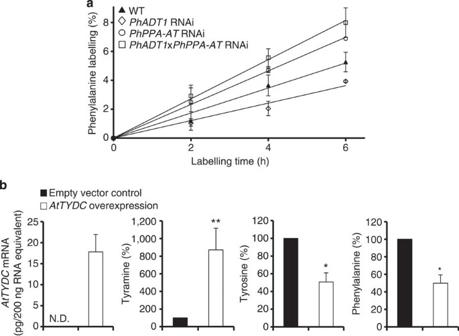Figure 5:In plantaevidence for the interconnection between tyrosine catabolism and phenylalanine biosynthesis. (a)15N-tyrosine labels phenylalanine in petunia flowers. 10 mM15N-tyrosine was fed to 2-day-old petunia flowers of WT (solid triangle), and thePhADT1(open diamond),PhPPA-AT(open circle) andPhADT1xPhPPA-AT(open square) RNAi lines for 2, 4 and 6 h beginning at 18:00 h. Labelling of phenylalanine pools were analysed by TOF LC-MS. Data are means±s.e.m. (n≥3 biological replicates except for thePhPPA-AT6-h time point,n=1). Incorporation of15N label in phenylalanine was linear over the 6-h time course (R2=0.9802, 0.9693, 0.9982 and 0.9977 for WT and thePhADT1,PhPPA-ATandPhADT1xPhPPA-ATRNAi lines, respectively). (b) Overexpression ofArabidopsis tyrosine decarboxylase (AtTYDC)decreases phenylalanine levels inPhADT1xPhPPA-ATRNAi petunia flowers. Levels ofAtTYDCmRNA, tyramine, tyrosine and phenylalanine in petunia flowers of thePhADT1xPhPPA-ATRNAi line infiltrated with agrobacterium carrying theAtTYDCconstruct (white bars) relative to an empty-vector control (black bars). Absolute transcript levels ofAtTYDCare shown as pg per 200 ng total RNA. Tyramine, tyrosine and phenylalanine levels are presented as a percentage relative to the corresponding empty-vector reference. Data are means±s.e.m. (n=3 biological replicates). *P<0.05 and **P<0.01 as determined by paired two-tailed Student’st-tests. N.D., not detectable. Figure 5: In planta evidence for the interconnection between tyrosine catabolism and phenylalanine biosynthesis. ( a ) 15 N-tyrosine labels phenylalanine in petunia flowers. 10 mM 15 N-tyrosine was fed to 2-day-old petunia flowers of WT (solid triangle), and the PhADT1 (open diamond), PhPPA-AT (open circle) and PhADT1 x PhPPA-AT (open square) RNAi lines for 2, 4 and 6 h beginning at 18:00 h. Labelling of phenylalanine pools were analysed by TOF LC-MS. Data are means±s.e.m. ( n ≥3 biological replicates except for the PhPPA-AT 6-h time point, n =1). Incorporation of 15 N label in phenylalanine was linear over the 6-h time course ( R 2 =0.9802, 0.9693, 0.9982 and 0.9977 for WT and the PhADT1 , PhPPA-AT and PhADT1 x PhPPA-AT RNAi lines, respectively). ( b ) Overexpression of Arabidopsis tyrosine decarboxylase (AtTYDC) decreases phenylalanine levels in PhADT1 x PhPPA-AT RNAi petunia flowers. Levels of AtTYDC mRNA, tyramine, tyrosine and phenylalanine in petunia flowers of the PhADT1 x PhPPA-AT RNAi line infiltrated with agrobacterium carrying the AtTYDC construct (white bars) relative to an empty-vector control (black bars). Absolute transcript levels of AtTYDC are shown as pg per 200 ng total RNA. Tyramine, tyrosine and phenylalanine levels are presented as a percentage relative to the corresponding empty-vector reference. Data are means±s.e.m. ( n =3 biological replicates). * P <0.05 and ** P <0.01 as determined by paired two-tailed Student’s t -tests. N.D., not detectable. Full size image To investigate whether the cytosolic pool of tyrosine can influence phenylalanine levels in vivo , the level of tyrosine was depleted in petunia flowers of PhADT1xPhPPA-AT RNAi via transient overexpression of the cytosolic Arabidopsis tyrosine decarboxylase (AtTYDC), which exclusively catalyses decarboxylation of L -tyrosine to tyramine [37] , [38] . AtTYDC overexpression resulted in 50% reduction of the tyrosine pool and a 9-fold increase in tyramine levels with a concomitant 50% decrease in phenylalanine levels ( Fig. 5b ). Recent investigations into aromatic amino-acid biosynthesis revealed that in contrast to most microbes, plants predominantly rely on the arogenate pathway to synthesize phenylalanine [15] , [16] , [17] , [18] . However, the results presented here demonstrate that downregulating PhPPA-AT in the PhADT1 RNAi background rescues phenylalanine and phenylalanine-derived volatile levels ( Fig. 2c , Supplementary Fig. S1 , and Supplementary Table S1 ), suggesting the redirection of carbon flux from prephenate via an alternative route and thus reopening de facto the search for plant genes participating in the microbial-like phenylpyruvate pathway ( Fig. 1 ). In this regard, a petunia aminotransferase, PhPPY-AT, which preferentially converts phenylpyruvate to phenylalanine and is unable to utilize prephenate as substrate ( Supplementary Table S3 ) was identified. Downregulation and overexpression of PhPPY-AT confirm the participation of PhPPY-AT in phenylalanine biosynthesis in vivo ( Fig. 4 and Supplementary Fig. S4 ), therefore establishing the existence of a functional alternative phenylpyruvate pathway in plants. Moreover, flux through the phenylpyruvate pathway is higher when the entry point into the arogenate pathway is blocked as it occurs in PhPPA-AT and PhADT1xPhPPA-AT RNAi lines ( Fig. 5a ). It still remains enigmatic why phenylalanine and phenylalanine-derived volatile levels in the PhADT1xPhPPA-AT RNAi line were completely restored to those of wild-type and not just to those of the PhPPA-AT RNAi line ( Fig. 2c , Supplementary Fig. S1 and Supplementary Table S1 ), despite identical metabolic profiles ( Supplementary Fig. S1 ) and comparable increases in flux through the phenylpyruvate pathway ( Fig. 5a ). The decreased flux in the PhADT1 RNAi line ( Fig. 5a ) is likely due to the overall reduction in phenylalanine biosynthesis via the downregulation of the upstream shikimate pathway [16] ( Supplementary Fig. S1 ). To date, it is believed that aromatic amino acids are exclusively synthesized in the plastid [10] , [16] , [18] , [29] , [30] , and then transported into the cytosol to serve as building blocks for proteins and precursors of downstream metabolites. In light of the absence of an N-terminal targeting signal and the confirmed cytosolic localization of PhPPY-AT ( Fig. 3 ), the all-plastidial paradigm of phenylalanine biosynthesis should be shifted to now include a cytosolic component ( Fig. 6 ). This discovery may also alter the already complex post-transcriptional regulatory model of carbon flux through the shikimate pathway, which involves feedback mechanisms controlled by phenylalanine levels in plastids [10] ( Fig. 6 ). Furthermore, it can be envisioned that this will influence future metabolic engineering strategies for manipulating production of numerous important plant products. 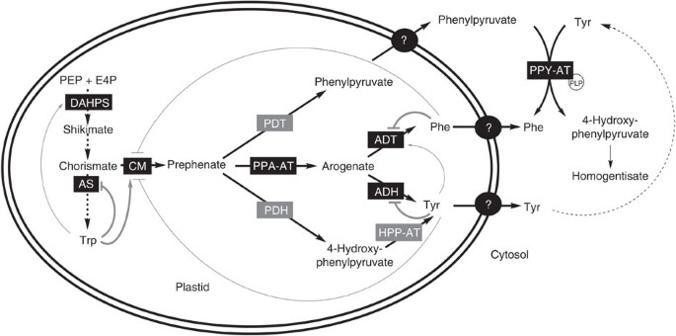Figure 6: Revised model for phenylalanine biosynthesis in plants. The new model for phenylalanine biosynthesis in plants now includes a cytosolic step linked to the catabolism of tyrosine, which is mediated by PPY-AT. Circles with question marks correspond to undefined transport steps, whereas grey lines depict activation and feedback inhibition with thickness indicating the relative strength of allosteric regulation. Known enzymes are shown with a black background, whereas those with a grey background are not yet characterized. ADH, arogenate dehydrogenase; ADT, arogenate dehydratase; AS, anthranilate synthase; CM, chorismate mutase; DAHPS, 3-deoxy-D-arabino-heptulosonate 7-phosphate synthase; E4P, D-erythrose 4-phosphate; HPP-AT, 4-hydroxyphenylpyruvate aminotransferase; PDH, prephenate dehydrogenase; PDT, prephenate dehydratase; PEP, phosphoenolpyruvate; PPA-AT, prephenate aminotransferase; PPY-AT, phenylpyruvate aminotransferase; Trp, tryptophan. Figure 6: Revised model for phenylalanine biosynthesis in plants. The new model for phenylalanine biosynthesis in plants now includes a cytosolic step linked to the catabolism of tyrosine, which is mediated by PPY-AT. Circles with question marks correspond to undefined transport steps, whereas grey lines depict activation and feedback inhibition with thickness indicating the relative strength of allosteric regulation. Known enzymes are shown with a black background, whereas those with a grey background are not yet characterized. ADH, arogenate dehydrogenase; ADT, arogenate dehydratase; AS, anthranilate synthase; CM, chorismate mutase; DAHPS, 3-deoxy-D-arabino-heptulosonate 7-phosphate synthase; E4P, D-erythrose 4-phosphate; HPP-AT, 4-hydroxyphenylpyruvate aminotransferase; PDH, prephenate dehydrogenase; PDT, prephenate dehydratase; PEP, phosphoenolpyruvate; PPA-AT, prephenate aminotransferase; PPY-AT, phenylpyruvate aminotransferase; Trp, tryptophan. Full size image The demonstration that phenylpyruvate serves as an intermediate in phenylalanine biosynthesis now implicates the existence of a functional prephenate dehydratase (PDT) converting prephenate to phenylpyruvate in plants ( Fig. 1 ). To date, PDT activity and phenylpyruvate have rarely been reported in plant tissues [16] , [39] . However, using triple quadrupole LC-MS we were able to detect PDT activity in petunia plastids and found it to be increased by approximately 2-fold in PhADT1xPhPPA-AT and parental RNAi lines ( Supplementary Fig. S5a ). Together with increased prephenate levels in the PhADT1xPhPPA-AT and PhPPA-AT RNAi lines ( Supplementary Fig. S1 ), these results suggest that increased PDT activity efficiently redirects carbon flux through the alternative phenylpyruvate route, resulting in elevated phenylalanine levels compared with the PhADT1 RNAi line ( Fig. 2c ). Although PDT activity also increased in the PhADT1 RNAi line, it is likely that carbon flux was not redirected through the phenylpyruvate route because prephenate failed to accumulate and flux through the shikimate pathway was reduced [16] ( Supplementary Fig. S1 ). It remains to be investigated if there is a dedicated PDT with strict specificity for prephenate catalysing this reaction, or if plants rely on one or more of the known ADTs that can use prephenate as substrate at low catalytic efficiencies [15] , [16] , [40] . In petunia, PhADT2 and PhADT3, but not PhADT1, are capable of utilizing prephenate [16] . However, their expression levels did not correlate with increased PDT activity in the arogenate pathway knockdown lines ( Supplementary Fig. S5b ), indicating either the participation of an unknown enzyme(s) or post-transcriptional upregulation of the aforementioned ADTs. Projecting forward, it is additionally necessary to understand how phenylpyruvate is transported out of the plastid to serve as substrate for the cytosolic aminotransferase ( Fig. 6 ). PhPPY-AT belongs to the class of tyrosine aminotransferases (EC 2.6.1.5) that are defined to catalyse the reversible conversion of tyrosine+2-oxoglutarate to 4-hydroxyphenylpyruvate+glutamate. Although tyrosine is the preferred amino donor for PhPPY-AT ( Supplementary Table S2 ), the unique property of this plant enzyme is that instead of 2-oxoglutarate serving as the primary keto acid acceptor, it preferentially uses phenylpyruvate ( Supplementary Table S3 ), thus suggesting an interconnection of the catabolism of tyrosine with the production of phenylalanine in the cytosol ( Fig. 6 ). The greater catalytic efficiency of the forward reaction (tyrosine+phenylpyruvate → 4-hydroxyphenylpyruvate+phenylalanine) over the reverse ( Table 1 ), as well as the impacts observed on the phenylalanine pool when PhPPY-AT expression is altered ( Fig. 4 ), further support such a relationship occurring in planta . The reduction in phenylalanine levels when the cytosolic tyrosine pool was depleted ( Fig. 5b ), together with the labelling retrieved in the amino group of phenylalanine from 15 N-tyrosine ( Fig. 5a ), provide direct in vivo evidence for the interconnection between these aromatic amino acids ( Fig. 6 ). It is foreseeable that PPY-ATs directly interconnecting tyrosine and phenylalanine metabolism are not limited to petunia. Further examination of the melon aromatic amino-acid aminotransferase, CmArAT1 (ref. 20 ), revealed that similar to PhPPY-AT, it also converts phenylpyruvate to phenylalanine ( Supplementary Table S4 ) using tyrosine as the preferred amino donor ( Supplementary Table S5 ). In addition, we observed that similar to petunia flowers ( Fig. 5a ), the phenylalanine pool in 5-week-old Arabidopsis inflorescence shoots was labelled by 4.16±0.23% after feeding 10 mM 15 N-tyrosine for 6 h. Moreover, a recent metabolic engineering study overexpressing PheA , a bacterial bifunctional chorismate mutase/PDT, in Arabidopsis plastids resulted in increased levels of phenylalanine and the tyrosine-derived metabolites homogentisate, tocopherols and tocotrienols [19] . Interestingly, homogentisate serves as the aromatic head group of the tocopherols and tocotrienols, and is synthesized in the cytosol from 4-hydroxyphenylpyruvate via tyrosine [5] ( Fig. 6 ). Although at the time the basis for the enhanced pools of tyrosine-derived metabolites in transgenic PheA Arabidopsis plants was unexplained [19] , in light of the current study, it is logical to suspect that increased flux from phenylpyruvate to phenylalanine drove that of tyrosine to 4-hydroxyphenylpyruvate via an aminotransferase orthologous to PhPPY-AT. Indeed, a Blastp search against Arabidopsis using PhPPY-AT as query retrieves as the best hit At5g53970, a recently characterized tyrosine aminotransferase demonstrated to be involved in tocopherol biosynthesis [23] . The discovery that the microbial-like phenylpyruvate pathway does in fact operate in plants raises many questions about the control of carbon flux towards phenylalanine and its downstream metabolites. One particularly crucial aspect that now must be taken into consideration is the role of compartmentalization and transport of intermediates in regulating flux through the phenylalanine biosynthetic pathways. It would also be interesting to explore the possibility of an analogous alternative pathway occurring for tyrosine biosynthesis from 4-hydroxyphenylpyruvate that a priori would be mediated by another aminotransferase ( Fig. 6 ). Finally, it should be emphasized that further studies are necessary to elucidate the functional relationship between the parallel pathways of phenylalanine biosynthesis, as well as that with tyrosine catabolism. Plant materials and metabolic analysis Petunia hybrida cv: Mitchell wild-type (Ball Seed Co., West Chicago, IL, USA) and transgenic PhADT1 RNAi, PhPPA-AT RNAi and crossed PhADT1 x PhPPA-AT RNAi plants were grown under standard greenhouse conditions [41] with a light period from 6:00 h to 21:00 h. Crossed lines were screened for the presence of transgenes by PCR on genomic DNA using gene-specific primers: forward 5′-GCTAAGCTGGAGTGCACATT-3′, and reverse 5′-ACCTGGTATGACCTTCACGA-3′ for PhPPA-AT and forward, 5′-ATTTCGAACAAGCGTACACC-3′ and reverse 5′ AATTGTGAGCGCCTTAGGTA-3′ for PhADT1 . Scent collection and targeted metabolic profiling of petunia petals were performed as described previously [16] , with the exception of scent collection time, which was from 18:00 h to 22:00 h. Gene expression analysis using qRT-PCR For RNA isolation, petals from at least eight petunia flowers were harvested at 20:00 h, 2 days after anthesis and immediately frozen in liquid nitrogen. Total RNA was isolated using an RNeasy plant mini kit (Qiagen, Valencia, CA, USA) and treated with DNase I to eliminate genomic DNA using the TURBODNA-free kit (Ambion, Foster City, CA, USA). One microgram of RNA was subsequently reverse-transcribed to cDNA in a total volume of 100 μl using the High Capacity cDNA reverse transcription kit (Applied Biosystems, Foster City, CA, USA). qRT-PCR analysis relative to the reference gene UBQ10 (ubiquitin 10) for PhADT1 , PhADT2 , PhADT3 , PhCM1 and PhPPA-AT were performed using gene-specific primer pairs ( Supplementary Table S6 ) [16] , [17] . Forward 5′-GCTTCTCACAAGTTCAATGGTTATGCT-3′ and reverse 5′-CCAGAAAGGCAATTGCAGATTATTT-3′ primers for PhPPY-AT were designed using PrimerExpress (Applied Biosystems, Foster City, CA, USA) and exhibited 93% efficiency at a final concentration of 500 nM. For absolute quantification of AtTYDC transcript levels, pCR4-TOPO vector carrying AtTYDC was digested with BamHI and EroRV and the resulting fragment was purified from agarose gel with a Qiaquick gel extraction kit (Qiagen, Valencia, CA, USA). Concentration of purified DNA fragment was determined with the NanoDrop 1000 spectrophotometer (Thermo Scientific, West Palm Beach, FL, USA). Several dilutions were prepared from 4 ng ml −1 to 6.4 pg ml −1 and used to obtain standard curves in qRT–PCR with gene-specific primers ( Supplementary Table S6 ) [38] . Individual qRT–PCR reactions contained 5 μl of the SYBR Green PCR master mix (Applied Biosystems, Foster City, CA, USA), 3 μl of 50-fold diluted cDNA, and 1 μl of 5 μM forward and reverse primers. Two-step qRT–PCR amplification (40 cycles of 95 °C for 3 s followed by 60 °C for 30 s) was performed using the StepOnePlus real-time PCR system (Applied Biosystems, Foster City, CA, USA). On the basis of the standard curves, absolute quantity of AtTYDC transcript was calculated and expressed as pg per 200 ng total RNA. Each data point represents an average of three to five independent biological samples with three technical replicates for each sample. Expression and purification of recombinant proteins For functional expression, the coding region of PhPPY-AT was amplified with forward 5′-CGCGCGGCAGCCATATGATGGAGACGAATGTGGTGAAAGTGA-3′ and reverse 5′-GTCATGCTAGCCATATGTCAACAGTGACCATTTTGTTGATATGAATG-3′ primers designed using the In-Fusion online tool ( http://bioinfo.clontech.com/infusion/convertPcrPrimersInit.do ). The amplified gene product was cloned into the NdeI site of pET28a containing an N-terminal (6xHis)-tag (Novagen, Madison, WI, USA) using In-Fusion cloning (Clonetech, Mountain View, CA, USA). For functional expression of CmArAT1 its coding region was obtained by PCR using forward 5′-AACATATGCATCATCATCATCATCACGAGATTGGAGCTGTGAAC-3′ and reverse 5′- GGATCCTTACAACATTAGTGTATGC-3′ primers with the pBK-CMV- CmArAT1 (ref. 20 ) as a template. The amplified gene product was cloned into a pET21a expression vector (Novagen, Madison, WI, USA) at the NdeI site with an N-terminal (6xHis)-tag. After sequence verification, recombinant PhPPY-AT and CmArAT1 were expressed in E. coli and purified on Ni-NTA resin (Qiagen, Valencia, CA, USA). Expression in E. coli Rosetta cells, induction, harvesting and crude extract preparation were performed as described previously [42] with the exception of lysis buffer, which contained 50 mM Tris-HCl (pH 7.5), 10 μM pyridoxal 5-phosphate (PLP), 5 mM β-mercaptoethanol, 300 mM NaCl and 10% glycerol. Fractions with the highest PPY-AT activity were desalted on the Sephadex G-50 Fine column (GE Healthcare Bio-Sciences AB, Uppsala, Sweden) into the buffer containing 20 mM Tris-HCl, pH 8.0, 1 mM EDTA and 10% glycerol and PLP was then added to 100 μM. 6xHis tag from purified protein was removed by thrombin (Sigma-Aldrich, St Louis, MO, USA) before biochemical and kinetic characterization of enzyme. Functional complementation of the E. coli mutant DL39 For functional complementation, the coding region of PhPPY-AT was obtained by PCR using forward 5′-CCGGGGATCCTCTAGAATGGAGACGAATGTGGTGAAAGTGA-3′ and reverse 5′-GCAGGTCGACTCTAGATCAACAGTGACCATTTTGTTGATATGAATG-3′ primers designed with the In-Fusion online tool. The amplified PhPPY-AT coding sequence was cloned into XbaI site of pBad33 (ref. 28 ) under control of an arabinose-inducible promoter using In-Fusion cloning and introduced into the DL39 mutant ( LAM-, aspC13, fnr-25, rph-1, ilvE12, tyrB507 ; Coli Genetic Stock Center, Yale University, New Haven, CT, USA) [27] , which is auxotrophic for phenylalanine, tyrosine, aspartic acid, valine, leucine and isoleucine. Functional complementation was performed essentially as described [21] . Starter cultures of wild-type E. coli K-12 and DL39 cells harbouring either empty pBad33 or the pBad33- PhPPYAT construct were grown in liquid M9 minimal medium containing 0.2% arabinose and 50 μg ml −1 phenylalanine, tyrosine, aspartic acid, valine, leucine and isoleucine. Chloramphenicol (25 μg ml −1 ) was also added to DL39 cells for plasmid selection. After 36 h of growth at 37 °C, cells were washed two times with M9 medium without antibiotics or amino acids, and resuspended to an OD 600 of 0.1, which was further used to create cell dilutions with an OD 600 of 1 × 10 −2 , 10 −3 and 10 −4 . Next, 5 μl of cells at each cell density were plated on M9 plates containing 0.2% arabinose and 50 μg ml −1 aspartic acid, valine, leucine and isoleucine, with and without 50 μg ml −1 phenylalanine and tyrosine. After 24 h at 37 °C, a positive functional complementation was assessed by looking for the restored ability of the DL39 mutant to grow in the absence of phenylalanine and tyrosine. Enzyme assays Recombinant PhPPY-AT activity was analysed in the reaction mixture (50 μl) containing 50 mM HEPES pH 10, 10 mM amino donor, 10 mM keto acid substrate and 200 μM PLP, which were preincubated at 30 °C for 5 min. The reaction was initiated by adding 5.6 μg of protein and incubated at 30 °C for 15 min. When Tyr was used as amino donor, 1.12 μg of protein was used and reactions were incubated for 3 min. For reverse reactions, 13.5 μg or 2.8 μg of enzymes were used for 4-hydroxyphenylpyruvate and α-ketoglutarate substrates, respectively. After termination of reaction with 50 μl of 1N HCl and centrifugation, 20 μl of the final reaction mixture was derivatized with o -phthalaldehyde and analysed by HPLC (Agilent 1200 HPLC system, Palo Alto, CA, USA) as described [17] . Plastidic PDT activity was analysed in the reaction mixtures (50 μl) containing 50 mM Na-phosphate (pH 8.0) and 3 mM prephenate, which were preincubated at 37 °C for 5 min. The reaction was initiated by adding 100 μg of plastidic protein and incubated at 37 °C for 60 min. The reaction was terminated by 50 μl of 100% MeOH. After protein precipitation, 10 μl of the final mixture was subjected to Triple Quadrupole LC-MS (Agilent 6460, Palo Alto, CA, USA). Chromatographic separation was performed using an Agilent 1200 LC system (Palo Alto, CA, USA) equipped with Atlantis dC18 column (3 μm, 150 × 2.1 mm; Waters, Milford, MA, USA) with a 20 min linear gradient of 0–95% acetonitrile in 1% formic acid. Phenylpyruvate was monitored in MRM (multiple reaction monitoring) mode and quantified based on a standard calibration curve generated with an authentic phenylpyruvate standard. The d 0 -phenylpyruvate data were acquired by monitoring the following transitions: 163.1→116.9 with a collision energy of 25 V, 163.1→100.9 with a collision energy of 25 V, and 163.1→91 with a collision energy of 5 V. The d 1 -prephenate data were acquired by monitoring the following transitions: 225→121 with a collision energy of 20 V, 225→109.1 with a collision energy of 10 V and 225→91.1 with a collision energy of 5 V. The dwell time for all data acquired was 50 ms and fragmentor voltage was 70 V. The jet stream ESI interface had a gas temperature of 325 °C, gas flow rate of 8 l min −1 , nebulizer pressure of 35 psi, sheath gas temperature of 250 °C, sheath gas flow rate of 7 l min −1 , capillary voltage of 3,000 V and nozzle voltage of 500 V. All enzyme assays were performed at an appropriate enzyme concentration so that reaction velocity was linear and proportional to enzyme concentration during the incubation time period. Kinetic data were evaluated by hyperbolic regression analysis (HYPER.EXE, Version 1.00, 1992). At least triplicate assays were performed for all data points. Preparation of plastidial and cytosolic fractions Plastids were isolated from 10 to 20 g of petals of 1–3 days old petunia flowers as described [43] . Petals were cut into small pieces, vacuum infiltrated twice for 3 min with chilled homogenizing buffer containing 0.5 M sorbitol, 20 mM HEPES/NaOH (pH 7.4), 10 mM KCl, 1 mM MgCl 2 .6H 2 O, 1 mM EDTA-Na 2 , 5 mM DTT, and 1% BSA and blended three times for 5 s in 200 ml of buffer. The homogenate was filtered through two layers of Miracloth (Calbiochem, La Jolla, CA, USA) and centrifuged at 2,500 × g for 5 min. The pellet was twice washed with 2 ml of 0.5 M sorbitol and 20 mM HEPES (pH 7.4), plastids were than resuspended in buffer containing 50 mM sodium phosphate buffer and 10% glycerol and used for enzyme assays. To prepare a cytosolic fraction, the remaining supernatant was centrifuged for an additional 20 min at 12,000 × g at 4C to pellet mitochondria and peroxisomes. The resulting supernatant (cytosolic fraction) was then concentrated and desalted into 50 mM sodium phosphate buffer and 10% glycerol using an Ultrafree-MC filter (Ultra-4; Millipore Amicon, Billerica, MA, USA ) before enzyme assays. Subcellular localization of PPY-AT Plasmid p326-sGFP containing the cauliflower mosaic virus 35S promoter was used for the generation of GFP fusion constructs. For the C-terminal GFP fusion (PhPPY-AT-GFP), the open reading frame of PhPPY-AT was amplified using forward primer 5′-GTCTAGAATGGAGACGAATGTGGTGAAAGTGA-3′, which introduced an XbaI site (underlined) upstream of ATG codon, and reverse primer 5′-CGGATCCACAGTGTGACCATTTTGTTGATATGAA-3′ containing a BamHI site (underlined). For the N-terminal GFP fusion (GFP-PhPPY-AT), the PhPPY-AT open reading frame was amplified by PCR using forward primer 5′-CTGTACAAGATGGAGACGAATGTGGTGAAAGTGA-3′, which introduced a BsrGI site (underlined) at the initiating ATG codon, in combination with reverse primer 5′-GGCGGCCGCTCAACAGTGACCATTTTGTTGATAT-3′, introducing a NotI site (underlined) after the stop codon. The PCR fragments were subcloned into the pGEM-T vector (Invitrogen, Carlsbad, CA, USA) and checked by sequencing for absence of errors during PCR amplifications. The XbaI-BamHI and BsrGI-NotI fragments were subcloned into the p326-sGFP vector in frame with GFP. Arabidopsis protoplasts were prepared and transformed as described previously [44] . The plasmids p326-sGFP and p326-RbTP-sGFP containing a plastidial Rubisco target peptide, were used as markers for cytosolic and plastidial localization, respectively. Transient expression of GFP fusion proteins was observed 16–20 h after transformation, and images were acquired using Zeiss LSM710 laser spectral scanning confocal microscope with a C-Apochromat 40 × /1.20 W objective (Zeiss, Thornwood, NY, USA). GFP was excited with an Argon laser at wavelength 488 nm and emissions were collected over a 493–598 nm bandpass. Chlorophyll fluorescence was excited by a HeNe laser at wavelength 633 nm and emissions were collected over a 647–721 nm bandpass. PhPPY-AT downregulation and overexpression in planta For the PhPPY-AT RNAi construct a synthetic DNA, containing two spliced PhPPY-AT cDNA fragments of the coding region corresponding to nucleotides 363–891 and 363–687, the latter in antisence orientation to form a hairpin structure, was synthesized (Genscript, Piscataway, NJ, USA). EcoRI and BamHI sites were introduced at the 5′ and 3′ ends during DNA synthesis and the resulting synthetic DNA fragment was subcloned into the EcoRI/BamHI site of pRNA69 vector containing LIS promoter [41] . Next, the part of constructed plasmid containing the LIS promoter and the two PPY-AT fragments in opposite orientation separated by the intron was cut out using SacI/NotI and subcloned into the pART27 simpler binary vector [45] . Transient PhPPY-AT downregulation was achieved using vacuum infiltration of at least 15 total 1-day-old petunia flowers from five different plants with Agrobacterium tumefaciens strain GV3101 containing pART27-LIS-PPY-AT RNAi and pART27-LIS vector (control) at OD 600 of 0.4 as described previously. Forty-eight hours after infiltration, scent was collected for 4 h from 18:00 h to 22:00 h and analysed by GC-MS [16] . For PhPPY-AT overexpression, the open reading frame of PhPPY-AT was amplified by PCR using forward 5′-CACCATGGAGACGAATGTGGTGAAAGTGA-3′ and reverse 5′-TCAACAGTGACCATTTTGTTGATATGAATG-3′ primers. The PCR fragment was subcloned into the pENTR/D-TOPO vector (Invitrogen, Carlsbad, CA, USA) and verified by sequencing for absence of errors during PCR amplifications. The Gataway cloning strategy was employed to subclone the PhPPYAT fragment into the destination vector pB2GW7 (Invitrogen, Carlsbad, CA, USA). Transient PhPPY-AT overexpression was performed as described previously [46] . AtTYDC overexpression in petunia flowers The Arabidopsis TYDC coding region was PCR-amplified using forward primer 5′-CCATGGATGGAATTTGGTACCGGCAACG-3′ and reverse primer 5′-TCCAAATTTACACGCAACGACCATTATTAACTGCAG-3′ and subcloned into the pGEMT easy vector (Invitrogen, Carlsbad, CA, USA). After sequence verification, the fragment was subcloned into the NcoI/PstI site of the pEF1-LIS binary vector [47] and transient AtTYDC overexpression was performed as described above. Labelling experiments Feeding experiments were performed as described previously [25] . Corollas from 2-day-old wild-type and transgenic petunia flowers were fed with 10 mM 15 N-Tyr,L-[ring- 2 H 4 ]-Tyr (Cambridge Isotope Laboratories, Andover, MA, USA), or L-[ring- 2 H 5 ]-Phenylpyruvate. L-[ring- 2 H 5 ]-Phenylpyruvate was synthesized by enzymatic conversion of L-[ring- 2 H 5 ]-Phe (Cambridge Isotope Laboratories, Andover, MA, USA) by melon CmArAT1 with a keto substrate α-ketoglutarate, and cofactor PLP. After filtration through an Ultrafree-MC filter and Dowex 50-H + × 8, 200 mesh column (Sigma-Aldrich, St Louis, MO, USA) to exclude proteins and amino acids, respectively, the purity of synthesized phenylpyruvate was analysed by TOF LC-MS and Triple Quadrupole LC-MS to ensure no contamination by labelled phenylalanine. Synthesized phenylpyruvate was 99.8% pure ( Supplementary Fig. S6 ) and used for feeding experiments. Tissues were collected after 2, 4 and 6 h for tyrosine, and after 6 h for phenylpyruvate, feeding starting at 18:00 h, followed by complete amino acid analysis as described previously [16] . The percentage of amino acid labelling was determined as the sum of the intensities of the shifted molecular ions divided by the sum of intensities for unshifted and shifted molecular ions, after correcting for natural isotope abundance. Accession code: PPY-AT sequence has been deposited in the NCBI Genbank nucleotide database under accession code KF511589 . How to cite this article: Yoo, H. et al . An alternative pathway contributes to phenylalanine biosynthesis in plants via a cytosolic tyrosine:phenylpyruvate aminotransferase. Nat. Commun. 4:2833 doi: 10.1038/ncomms3833 (2013).